Polarization maintaining single-mode low-loss hollow-core fibres Hollow-core fibre (HCF) is a powerful technology platform offering breakthrough performance improvements in sensing, communications, higher-power pulse delivery and other applications. Free from the usual constraints on what materials can guide light, it promises qualitatively new and ideal operating regimes: precision signals transmitted free of nonlinearities, sensors that guide light directly in the samples they are meant to probe and so on. However, these fibres have not been widely adopted, largely because uncontrolled coupling between transverse and polarization modes overshadows their benefits. To deliver on their promises, HCFs must retain their unique properties while achieving the modal and polarization control that are essential for their most compelling applications. Here we present the first single-moded, polarization-maintaining HCF with large core size needed for loss scaling. Single modedness is achieved using a novel scheme for resonantly coupling out unwanted modes, whereas birefringence is engineered by fabricating an asymmetrical glass web surrounding the core. The discovery of bandgap guided fibres [1] radically changed the rules of what kinds of materials could guide light. Most dramatically, bandgap-guided hollow-core fibres (HCFs) can guide light in materials like air or water, even though their refractive index is lower than any available solid cladding material [2] , [3] , [4] , [5] . The unique, qualitative advantages of HCFs seem perfectly suited to many applications: In data transmission and precision measurement, ultra-low nonlinearity removes a key fundamental limit on signal-to-noise ratio. In sensing of gas and liquid samples, low-loss guidance directly in the sample provides ideal sensitivity. In delivery of high-power pulses, guidance in air avoids damage of the core material. In low-latency transmission, guidance in air provides the guaranteed lowest time-of-flight delay possible. Despite these unique, qualitative benefits, and many exciting laboratory demonstrations [6] , [7] , [8] , [9] , [10] , [11] , [12] , HCF have so far not been widely adopted for use in real applications. This is largely because they are few-moded and have the awkward combination of poor polarization holding with high-polarization mode dispersion. Poor modal and polarization control make it difficult to fully utilize their benefits: for example, ultra-low nonlinearity is a clear advantage in applications requiring very precise interferometric sensing, but in these applications noise arising from polarization drift and coupling between transverse modes could easily degrade precision, and outweigh the benefit of low nonlinearity. There is a fundamental difficulty in achieving modal or polarization control in a low-loss HCF. Scattering losses are minimized by increasing the core size and reducing the interaction of light with the surface of glass webs surrounding the core [13] . But a large core typically means that unwanted modes are well guided—making the fibre less single-moded [14] . Further, light that does not interact with the glass tends not to see any intentional asymmetry–making it difficult to achieve substantial birefringence with losses less than around 10 dB km −1 (ref. 15 ). Introducing stress in the core (the dominant method of making conventional, solid polarization-maintaining (PM) fibres) is clearly not possible in a hollow fibre. Thus, birefringence must be achieved by carefully controlling the asymmetry of glass webs around the core [16] , [17] , such that surface mode interactions shift one polarization relative to the other. As these surface mode interactions can provide suppression of higher-order modes (HOMs) in narrow wavelength ranges, this strategy has even resulted in simultaneous polarization-maintenance and single-modedness [18] , [19] in small-core fibres. These results are difficult to extend to larger core size without design features that specifically control HOM suppression. Despite this fundamental tradeoff between birefringence and loss, we achieved excellent polarization properties: polarized light propagating through 467 m of fibre maintains a well-controlled polarization, with extinction ratio 32 dB. We have thus demonstrated beat lengths and extinction ratios typical of commercial solid-core fibres with stress rods, even though hollow-core guidance precludes strain-induced birefringence. Polarization control was obtained through a combination of birefringence (which limits coupling) and polarization dependent loss (PDL) (which suppresses any light that is coupled out of the desired polarization). We have simultaneously achieved single-modedness by introducing hollow ‘shunt’ features in the cladding, so that unwanted modes are coupled to the shunts and stripped away. We use a novel variation [20] on resonant-coupling [21] , [22] : perturbed resonance for improved single-modedness (PRISM). This scheme utilizes random bend-induced perturbations to make the resonance condition immune to fabrication imperfections, thus allowing robust single-modedness despite the intrinsic sensitivity of HCFs. Results presented here demonstrate that this mechanism is indeed sufficiently robust to allow fibres with additional design complexity needed for polarization control. Fabricated fibre The fibre shown in scanning electron microscope image ( Fig. 1a ) achieves excellent polarization control through tiny asymmetries in its geometry. The fibre was produced using the stack-and-draw technique. Although the geometry is suggestive of the traditional stress-rod structure of the solid PM fibres, this is a false analogy: the two hollow seven-cell shunts are included in the cladding in order to selectively suppress HOMs of the core. They are not an effective way to produce strong polarization dependence, as we have confirmed with various simulations and measurements. The fundamental modes in a low-loss 19-cell HCF are very well confined to the core, and see very little beyond the first layer of cladding holes. Polarization dependence was produced by a tiny variation in the thickness of the core wall with angle: a birefringent axis is defined by a core web that is thicker on the axis perpendicular to the shunts (top and bottom of the core as shown in Fig. 1a ), difficult to make out in the image. This is accomplished by using thick-walled capillaries: at the two top and two bottom positions adjacent to the core, capillaries have 60% larger cross-sectional glass area than the other lattice capillaries. The inner cladding consists of a lattice of air holes spaced L =5.0 μm apart, with silica webs and an air-fill-fraction around 95%, so that the lattice web thickness is estimated to be around 90 nm. The central core has diameter 26.0 μm, slightly above the D core ~5 L expected for a core of the 19-cell type (the core spans 19 lattice cells). The diameter of each shunt is around 13.3 μm. The nominal core web thickness is estimated to be around 2.3 times the thickness of a lattice web, whereas the shunt webs are around 1.4 times that of a lattice web. 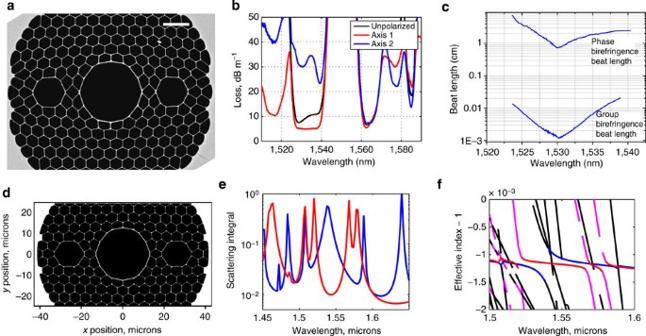Figure 1: Demonstration of polarization control in a hollow-core fibre. (a) A scanning electron microscope microscope image shows the geometry of the PM PRISM fibre (scale bar indicates 10 microns). (b) Measured loss for the two polarizations shows multiple low-loss windows, including one with large broadband polarization-dependent loss useful for suppressing the unwanted polarization. (c) Measured phase birefringence and group birefringence are plotted as beat lengths, demonstrating a minimum beat length below 7 mm. (d) Simulations illustrate the surface-mode coupling mechanism for a geometry roughly analogous to the measured fibre. (e) A surface mode crossing at 1,540 nm causes large scattering in one polarization (blue) but not the other (red). (f) Effective index displays the characteristic anti-crossing behaviour for the coupled polarization (blue). Surface modes are shown in black, except for those of the same symmetry class as the low-loss signal mode (pink), which have no crossing near 1,540 nm. Figure 1: Demonstration of polarization control in a hollow-core fibre. ( a ) A scanning electron microscope microscope image shows the geometry of the PM PRISM fibre (scale bar indicates 10 microns). ( b ) Measured loss for the two polarizations shows multiple low-loss windows, including one with large broadband polarization-dependent loss useful for suppressing the unwanted polarization. ( c ) Measured phase birefringence and group birefringence are plotted as beat lengths, demonstrating a minimum beat length below 7 mm. ( d ) Simulations illustrate the surface-mode coupling mechanism for a geometry roughly analogous to the measured fibre. ( e ) A surface mode crossing at 1,540 nm causes large scattering in one polarization (blue) but not the other (red). ( f ) Effective index displays the characteristic anti-crossing behaviour for the coupled polarization (blue). Surface modes are shown in black, except for those of the same symmetry class as the low-loss signal mode (pink), which have no crossing near 1,540 nm. Full size image Polarization control through surface mode engineering Polarization control is achieved by harnessing the very surface modes that normally degrade the performance of HCFs. These are the modes localized at the core web, and so they very effectively sample the asymmetry in the core web. They are a central part of understanding HCF because they couple strongly with core modes at any wavelength where they are phase-matched [23] . Much effort has focused on eliminating these phase-matching points, as they generally lead to high loss and reduced bandwidth. For a well-designed asymmetry, however, the surface modes can be highly birefringent [15] , [16] , [17] , [18] , [19] . Core modes of the two polarizations can see phase-matched coupling at different wavelengths. This means that at the signal wavelength, one polarization mode experiences strong surface-mode coupling and loss, whereas the other mode remains well guided. The measured loss in Fig. 1b illustrates this behaviour, showing loss measured by cutback in a 500-m section of fibre: light polarized along one polarization (axis 2) observes strong surface-mode features at 1,535 and 1,537 nm resulting in loss peaks at these wavelengths and substantial loss throughout this band (wavelengths below ~1,560 nm). Light launched along axis one instead sees only a narrow surface-mode peak at 1,524 nm, and so has a window of low-loss (<10 dB km −1 ) operation from 1,526 to 1,540 nm, with a minimum loss of 4.9±0.6 dB km −1 . The birefringent beat length was measured, with a minimum below 6 mm; remarkably, this low-loss HCF achieves beat length in the range of commercial PM fibres, even though the usual mechanism (stress) is not available. That figure also highlights the dramatic difference between phase and group birefringence for these structures, with nearly three orders of magnitude difference in measured beat length. The physics underlying this performance is illustrated by simulations of Fig. 1e,f . These do not attempt to reproduce the detailed measurement results, as intrinsic sensitivity and limits of precisely fabricating or characterizing a HCF geometry generally prohibit this [24] , [25] . Instead, simulations focus on qualitative agreement using an idealized version of the measured geometry ( Fig. 1d ), including a similar distortion pattern of the cladding. Figure 1e shows surface scattering (proportional to loss [13] ) for the two polarizations, and has a shape qualitatively similar to the measured loss (where the low-loss high-PDL window is at 1,540 nm for the calculation). Notably, the polarization properties are completely different for different low-loss wavelength bands (1,540 and 1,600 nm) as the mechanism for polarization dependence is a resonant effect, analogous to the measured results. Figure 1f shows the effective index, with a clear anti-crossing for the high-loss polarization, characteristic of resonant coupling: as wavelength is varied past the phase-matching point (1,540 nm), the core mode with this polarization (blue) continuously transforms into a surface mode (black). The curve is thus pulled away from that of the low-loss polarization (red). Interaction with the surface mode thus produces large calculated birefringence Δ n eff =3 × 10 −4 (beat length ~5 mm). Interestingly, the plot shows several surface mode crossings with various degrees of polarization dependence, only one of which leads to large birefringence. Polarization maintenance at an anti-crossing Clear evidence of an anti-crossing around 1,530 nm is contained in the measured interference between the two polarizations ( Fig. 2 ). When both polarizations are excited, their interference as a function of wavelength ( Fig. 2a ) is used to extract the group birefringence of Fig. 1c , or equivalently the differential group delay (DGD). Normally, the fringes would be analysed as beating between two modes, with negligible impact from any other modes of the fibre. However, the spectrogram analysis in Fig. 2b illustrates multiple beat notes: there is not only a ‘slow’ beating between the two core modes (for example, 25 ps delay over 40 cm fibre length at 1,525 nm), but also a much faster beating between a core mode and another (surface) mode (for example, 275 ps delay at 1,525 nm). As the resonant wavelength is passed, the high-loss core mode continuously transforms into the surface mode and vice-versa. Beating with the low-loss polarization, shown by the two traces in the sliding window plot ( Fig. 2b ), likewise takes the form of a continuous transformation: the fast and slow beating become less distinct and eventually cross at the wavelength of highest polarization-dependent loss. S 2 imaging measurements [26] , [27] , [28] were performed to confirm the nature of the modes seen in the spectrogram, and the measured mode images are also shown in Fig. 2b . 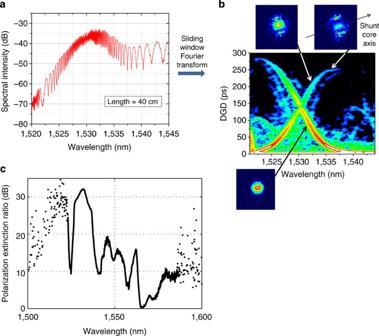Figure 2: Measured polarization beating and purity. (a) Beating between polarizations reveals two distinct Fourier components (b), as the low-loss polarization interferes with a modal mixture: the high-loss polarization is coupled to a surface mode. The beat notes show a transition of core mode to surface mode as wavelength is varied across the phase-matched resonance, confirmed by mode images obtained from an S2imaging measurement. (c) The fibre allows highly pure polarization to be transmitted over long lengths, as shown by the 32 dB extinction ratio measured after 467 m of fibre. Figure 2: Measured polarization beating and purity. ( a ) Beating between polarizations reveals two distinct Fourier components ( b ), as the low-loss polarization interferes with a modal mixture: the high-loss polarization is coupled to a surface mode. The beat notes show a transition of core mode to surface mode as wavelength is varied across the phase-matched resonance, confirmed by mode images obtained from an S 2 imaging measurement. ( c ) The fibre allows highly pure polarization to be transmitted over long lengths, as shown by the 32 dB extinction ratio measured after 467 m of fibre. Full size image The fibre’s high birefringence and polarization-dependent loss enable transmission of a well-controlled polarization over long lengths of fibre. The measured PER after 467 m of fibre is shown in Fig. 2c , reaching 32 dB at 1,532 nm. This exceeds the specification required for many PM fibre applications. Engineering the core web asymmetry produces surface modes localized along the access of asymmetry, and thus enables control of the birefringence resulting from surface mode coupling. Log-scale intensity plots for the calculated modes are shown for the low-loss (i) and high-loss polarization (ii), showing the strong component localized at the thick webs (top and bottom of the core) at the wavelength of highest PDL. Measured near-field images ( Fig. 3c–h ) are remarkably similar, confirming that the polarization-dependence achieved is a direct result of the controlled asymmetry designed into the structure. Images of the high-loss polarization ( Fig. 3d,e ) at high-PDL wavelengths show bright spots at the location where core webs are thicker, whereas the low-loss polarization shows essentially no intensity in this region. As expected, this effect is much less pronounced at 1,562 nm, where polarization-dependent loss is low. 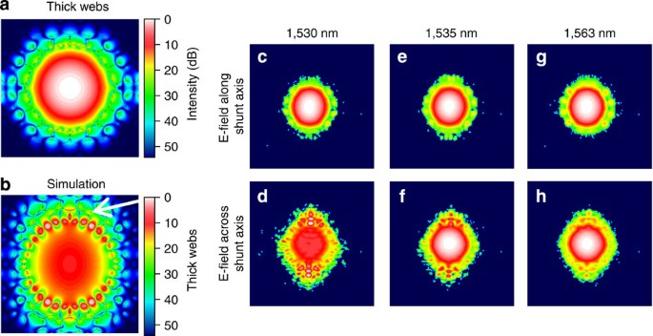Figure 3: Engineered surface modes. (a,b) Simulated mode intensities show that the high-loss polarization strongly interacts with the thick webs at the top and bottom of the core (indicated by white arrow), whereas the low-loss polarization interacts very little with glass webs, consistent with its low loss. Measured near-field profiles (c–h) strongly resemble calculated mode images. The same dB-scale colourmap was used for measurements and simulations. Figure 3: Engineered surface modes. ( a , b ) Simulated mode intensities show that the high-loss polarization strongly interacts with the thick webs at the top and bottom of the core (indicated by white arrow), whereas the low-loss polarization interacts very little with glass webs, consistent with its low loss. Measured near-field profiles ( c – h ) strongly resemble calculated mode images. The same dB-scale colourmap was used for measurements and simulations. Full size image The same fibre also represents a large step towards fulfilling the promise of PRISM fibres. The first published PRISM fibre results showed that this approach could simultaneously achieve lower loss and much better single-modedness than any seven-cell fibre, thus breaking the tradeoff between loss and modal control. However, the actual loss reported (7.5 dB km −1 at 1,590 nm) was still significantly higher than the record [13] for larger-core HCF (1.2 dB km −1 in a 19-cell core). The current results close part of this gap, showing that a single-moded PRISM fibre can achieve loss below 5 dB km −1 , even while meeting the conflicting challenge of operating in a high-PDL regime (which comes with an additional and significant loss mechanism of polarization cross-coupling). Modelling and experimental results so far suggest that including shunts does not increase the loss relative to a single-core fibre with the same core geometry, and so we are optimistic that lower loss will be achieved in future PRISM fibres. The PRISM strategy is a robust adaptation of resonantly coupled fibre design, which does not require that the fabricated fibre geometry provide perfectly resonant coupling of all unwanted core modes [16] . Small index mismatches between a higher-order core mode and shunt modes will intermittently be cancelled by the bend-induced index tilt [29] , [30] , [31] , as long as the fibre is bent tightly enough and the orientation of the fibre with respect to the bend is allowed to drift, as shown schematically in Fig. 4a . These intermittent resonances provide suppression of the HOMs over only a fraction of the total fibre length, but are sufficient to achieve single-moded operation. 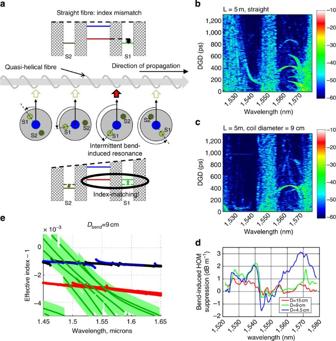Figure 4: Unwanted modes stripped by PRISM fibre. A PRISM fibre suppresses higher-order core modes that have small effective index mismatch compared with shunt modes (a). Bending the fibre introduces an index tilt that varies as the orientation drifts. This occasionally cancels the index mismatch, so that the modes experience intermittent coupling. Measured modal interference (b,c) shows moderate mode content for straight fibre near 1,530 nm, but this is drastically reduced when the fibre is coiled to 9 cm diameter. From the reduction in modal interference, HOM suppression >1 dB m−1is estimated (d). The need for coils of this rough size is generally consistent with effective index calculations (e); the mismatch between shunt modes (dark green) and LP11-like modes (red) can be cancelled if the shunt modes are perturbed by bends of diameter 9 cm (light green). Here, both fundamental modes are shown in blue. Figure 4: Unwanted modes stripped by PRISM fibre. A PRISM fibre suppresses higher-order core modes that have small effective index mismatch compared with shunt modes ( a ). Bending the fibre introduces an index tilt that varies as the orientation drifts. This occasionally cancels the index mismatch, so that the modes experience intermittent coupling. Measured modal interference ( b , c ) shows moderate mode content for straight fibre near 1,530 nm, but this is drastically reduced when the fibre is coiled to 9 cm diameter. From the reduction in modal interference, HOM suppression >1 dB m −1 is estimated ( d ). The need for coils of this rough size is generally consistent with effective index calculations ( e ); the mismatch between shunt modes (dark green) and LP11-like modes (red) can be cancelled if the shunt modes are perturbed by bends of diameter 9 cm (light green). Here, both fundamental modes are shown in blue. Full size image Strong suppression of HOMs is experimentally confirmed in Fig. 4b–e . Mode content is quantified by analysing modal interference [16] , [26] , [27] , [28] , which can be plotted as a function of wavelength and delay in the sliding-Fourier maps of Fig. 4b,c . There is substantial interference with unwanted mode in the wavelength range of interest when the fibre is straight, but this mode content is greatly reduced when the fibre is coiled to 9 cm diameter or tighter. Bend-induced loss can be inferred by comparing the total HOM content from Fig. 4b,c , and is plotted in Fig. 4d , showing ~dB m −1 loss for D bend ≤9 cm in the wavelength range of interest (values around 1,550 nm wavelength are outside of the low-loss windows, and should be regarded as noise). Although no optical fibre is ever rigorously single-moded (even standard ‘single-mode fibres’ have cladding modes), the level of suppression we have measured will make these fibres effectively single-moded for many applications. For comparison, in telecommunications, the standard ‘cable cutoff’ definition is defined by propagation through 22 m of fibre in a combination of 8 and 28 cm coil diameters. HOM loss of 1–2 dB m −1 is consistent with strongly suppressing unwanted modes in ~22 m of fibre. The PRISM fibre presented here would require somewhat tighter bends than commercial telecom fibres, but 9 cm diameter bending should be achievable through proper cable design. Likewise, for other potential applications, the fibre will show effectively single-mode behaviour as long as all relevant lengths (total length, length between splices, etc) are ~10 m or greater, so that light accidentally launched in the HOMs is substantially removed. Although cabling, connectorization and other practical issues require further investigation, progress in these areas (for example, low-loss low-reflection ‘mechanical splices’ [32] ) is very encouraging. We have demonstrated a 500-m-long PM and single-transverse-mode HCF with loss within a few times of the record for any HCF. For many applications, this means that the unique game-changing advantages of HCF (for example, low-nonlinearity) are no longer hypothetical: these fibres have the modal and polarization control needed to be incorporated into high-performance systems. These results also demonstrate that fabrication advances and robust fibre design principles now allow HCFs much more complex than the usual ‘step index’ designs: realistic HCFs can utilize advanced design features to achieve seemingly conflicting requirements. Simulations Numerical calculations were done with a 2d finite difference vector mode solver [33] . Geometrical parameters were determined from microscope images, but were also adjusted within the range of measurement uncertainties to fit optical measurements, for example, the lattice air-fill-fraction for the simulation was set to 95.0% to match the bandgap position. Fibre measurements Measurements of group birefringence were obtained from spectral interference of the form shown in Fig. 2a . Bulk optic polarizers at the input and output of the fibre were aligned to maximize the observed spectral interference. The output beam was focused onto a single-mode fibre that was coupled to an optical spectrum analyser with 0.01 nm resolution bandwidth. Phase birefringence measurements were obtained by cutting back the length of the fibre under test in small increments and measuring the group birefringence beating as a function of the length. As the fibre was cutback, the power at any given wavelength oscillated between maxima and minima. The phase birefringence beat length at that wavelength was the length fibre to go from one minima to the next. Cutbacks as short as 0.5 mm in length were performed to ensure that the cutback length was much shorter than the minimum phase birefringence beat length. The images of the HOMs in the PM spectrogram of Fig. 2b were obtained using S 2 imaging, which is based on coherent interference of multiple modes co-propagating in the HCF. Light from a narrow linewidth tunable laser was launched into the fibre under test using bulk-optic coupling. The output of the HCF was flat cleaved and the beam launched into free space. Input and output polarizers were aligned to maximize the spectral interference because of polarization beating, such as that observed in Fig. 2a . The beam was imaged onto an InGaAs camera sensitive at 1,550 nm. The beam profile of the fibre under test was obtained, as the wavelength of the narrow linewidth laser was tuned. HOM images and relative power levels were obtained via the data analysis described in ref. 27 . The sliding Fourier window calculation of HOM spectrograms is based on measuring interference between coherent modes that propagate with different group delays in the fibre under test [10] , [19] . The input and output of 5 m lengths of HCFs were fusion spliced to standard single-mode fibre. The fusion splice was made as short and cold as possible to prevent the collapse of holes in the HCF. Note that because there are two SMF-HCF splices in the experiment, with each splice acting as a mode transformer, the mode content transmitted through the system is approximately half the mode content propagating in the HCF. A narrow linewidth (few hundred kHz) tunable laser was launched into the fibre under test, and the transmission was measured with a power metre. The frequency of the laser was tuned through the wavelength range of interest. The maximum tuning range of the laser was 1,500–1,610 nm, and the step size was 0.003 nm. A small subset of the transmission data with a width of approximately 3 nm was selected with a narrow window and Fourier-transformed. The window is then slid through the entire transmission spectrum. The data analysis of ref. 28 relating Fourier transform amplitude to mode amplitude was then applied, to produce a plot of mode content vs wavelength and group delay. Because the modes are co-propagating, the modes are measured as a function of differential group delay, or difference in group delay between the fundamental mode and the HOMs. How to cite this article: Fini, J. M. et al . Polarization maintaining single-mode low-loss hollow-core fibres. Nat. Commun. 5:5085 doi: 10.1038/ncomms6085 (2014).